Amine synthesis via iron-catalysed reductive coupling of nitroarenes with alkyl halides (Hetero)Aryl amines, an important class of organic molecules in medicinal chemistry, are most commonly synthesized from anilines, which are in turn synthesized by hydrogenation of nitroarenes. Amine synthesis directly from nitroarenes is attractive due to improved step economy and functional group compatibility. Despite these potential advantages, there is yet no general method for the synthesis of (hetero)aryl amines by carbon–nitrogen cross-coupling of nitroarenes. Here we report the reductive coupling of nitroarenes with alkyl halides to yield (hetero)aryl amines. A simple iron catalyst enables the coupling with numerous primary, secondary and tertiary alkyl halides. Broad scope and high functional group tolerance are demonstrated. Mechanistic study suggests that nitrosoarenes and alkyl radicals are involved as intermediates. This new C–N coupling method provides general and step-economical access to aryl amines. Amines are among the most important organic compounds for the chemical, materials, pharmaceutical and agrochemical industries [1] , [2] , [3] . In particular, aromatic and heteroaromatic amines occupy a privileged position in the medicinal chemistry [3] , [4] , as exemplified in the top-selling drugs such as Abilify, Crestor, Gleevec and Lidoderm [5] . The most general methods to prepare aryl and heteroaryl amines are amine-carbonyl reductive amination [6] ( Fig. 1a ), direct alkylation of amines with alkyl halides [7] ( Fig. 1b ), and Buchwald–Hartwig [8] , [9] , [10] and Ullman-type carbon–nitrogen (C–N) cross-coupling reactions [11] , [12] ( Fig. 1c ). These amination methods employ amines, especially anilines, as the nitrogen source, which are usually prepared in advance by the hydrogenation of nitroarene derivatives [13] . Amine synthesis using directly nitro(hetero)arenes is attractive as it eliminates the hydrogenation step, saving time and cost. Moreover, functional groups such as amine, hydroxyl and thiol have orthogonal reactivity to the nitro group, so they may be tolerated without protection [14] . On the contrary, in amine synthesis using anilines, these groups have to be protected to avoid undesirable alkylation or arylation [14] . Recently, Baran and co-workers [14] developed a novel and elegant hydroamination approach to synthesize (hetero)aryl amines from nitro(hetero)arenes and olefins using an iron salt as catalyst, phenylsilane as hydrogen donor, and zinc (Zn) as reductant ( Fig. 1d ). Nevertheless, this approach was mostly efficient for the synthesis of (hetero)aryl amines substituted by a tertiary alkyl group [15] . General methods for amine synthesis from nitroarenes remain underdeveloped despite their potential advantages [14] , [16] , [17] . 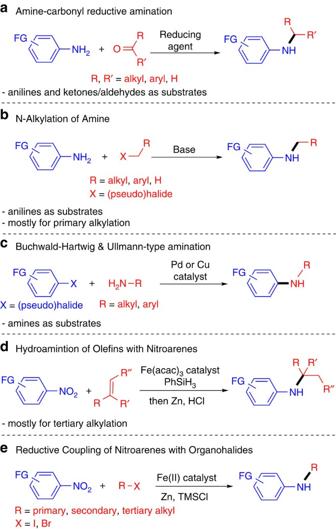Figure 1: Different approaches to (hetero)aryl amines. (a) Reductive amination; (b)N-Alkylation of amine; (c) Buchwald–Hartwig and Ullmann-type coupling; (d) Baran’s hydroamination with nitro(hetero)arenes; (e) Current work using reductive coupling of nitro(hetero)arenes with alkyl halides. Fe(acac)3, iron(III) acetylacetonate; PhSiH3,phenylsilane; Zn, zinc; TMSCl, chlorotrimethylsilane. Figure 1: Different approaches to (hetero)aryl amines. ( a ) Reductive amination; ( b ) N -Alkylation of amine; ( c ) Buchwald–Hartwig and Ullmann-type coupling; ( d ) Baran’s hydroamination with nitro(hetero)arenes; ( e ) Current work using reductive coupling of nitro(hetero)arenes with alkyl halides. Fe(acac) 3 , iron(III) acetylacetonate; PhSiH 3 ,phenylsilane; Zn, zinc; TMSCl, chlorotrimethylsilane. Full size image Here, we report (hetero)aryl amine synthesis via iron-catalysed reductive coupling of nitro(hetero)arenes with alkyl halides ( Fig. 1e ). This single-step cross-coupling approach allows the liaison to various types of carbon groups. Indeed, not only tertiary alkyl halides, but also secondary and primary alkyl halides could be coupled. The method tolerates a large number of functional groups, including those that require protection under conventional amine synthesis. Reaction design We recently reported Fe-catalysed reductive coupling of terminal aryl alkynes with non-activated alkyl halides to give cis -olefins [18] . Mechanistic study suggested that alkyl radical was involved as an intermediate, which added to terminal alkyne to form the C–C bond. Inspired by Baran’s proposal that alkyl radical could add to nitrosoarene, formed by the reduction of nitroarene [14] , we envisioned that reductive coupling of nitroarenes and alkyl halides might be used to form secondary alkyl aryl amines according to the following pathways ( Fig. 2 ): an iron(II) precatalyst (Fe(II)) is reduced by zinc to Fe(I) (refs 18 , 19 , 20 ; Fig. 2a ), which is then able to activate an alkyl halide to give an alkyl radical and regenerate Fe(II) (ref. 18 ; Fig. 2b ). Meanwhile, nitroarene is reduced by zinc to form nitrosoarene [21] , [22] ( Fig. 2c ). The alkyl radical attacks the nitrogen atom of nitrosoarene to form the C–N bond [14] , and reduction of the resulting intermediate by zinc in the presence of an oxophilic Lewis acid such as chlorotrimethylsilane (TMSCl) shall give the amine product ( Fig. 2c ). 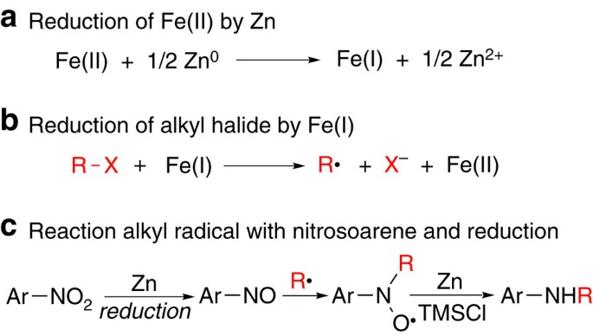Figure 2: Mechanistic design for Fe-catalysed reductive coupling of nitroarene with alkyl halide. (a) Reduction of iron(II) to iron(I); (b) activation of alkyl halide by iron(I); (c) reaction of alkyl radical with nitrosoarene and subsequent reduction to give alkyl aryl amine. ArNO2, nitroarene; RX, alkyl halide; TMSCl, chlorotrimethylsilane. Figure 2: Mechanistic design for Fe-catalysed reductive coupling of nitroarene with alkyl halide. ( a ) Reduction of iron(II) to iron(I); ( b ) activation of alkyl halide by iron(I); ( c ) reaction of alkyl radical with nitrosoarene and subsequent reduction to give alkyl aryl amine. ArNO 2 , nitroarene; RX, alkyl halide; TMSCl, chlorotrimethylsilane. Full size image Screening of reaction conditions We commenced the study by examining the reaction of nitrobenzene ( 1a ) with 2-iodooctane ( 2a ) ( Supplementary Tables 1–9 ). After a screening of reaction parameters, we found that the optimized conditions involved the use of N -methylpyrrolidone (NMP) as solvent, iron(II) chloride tetrahydrate (FeCl 2 ·4H 2 O) as catalyst (20 mol%), Zn (3 equiv.) as reductant, and TMSCl (2 equiv.) as co-reductant. The optimal loading of 2-iodooctane was 3 equiv. The reaction completed after 16 h at 90 °C. After an acidic workup, N -(2-octyl)aniline ( 3a ) was obtained in a nearly quantitative yield without over-alkylation ( Supplementary Table 9 , entry 1). Among various iron salts, FeCl 2 ·4H 2 O was the best catalyst ( Supplementary Table 1 , entries 1–16). When FeCl 2 ·4H 2 O was replaced by catalysts based on copper, cobalt, nickel, manganese, chromium, palladium and silver, the yields were lower ( Supplementary Table 1 , entries 17–29). When 99.99% pure FeCl 2 ·4H 2 O was used, the yield was similar ( Supplementary Table 8 , entry 3). Without TMSCl but under otherwise optimal conditions, the yield was 73% ( Supplementary Table 9 , entry 3). Substrate scope of secondary and tertiary alkyl halides The above conditions proved to be general for the coupling of various nitro(hetero)arenes and secondary and tertiary alkyl halides ( Fig. 3 ). The protocol is insensitive to the electronics of nitroarenes, as nitrobenzene ( 3a ) and its derivatives containing electron-withdrawing ( 3b - 3e, 3i – 3p, 3r ) or electron-donating groups ( 3f, 3g, 3q, 3s – 3v, 5b, 5u ) all reacted to yield the corresponding secondary aryl amines in synthetically useful yields. Functional group such as trifluoromethoxy ( 3b ), aryl bromo ( 3c ), aryl chloro ( 3d ), aryl iodo ( 3i ), nitrile ( 3e ), olefin ( 3h ), alkyne ( 3n ), ester ( 3k, 3l ), keto ( 3m ) and thiomethyl ( 3o ) were all tolerated. Thanks to the orthogonal reactivity of nitro groups with protic functional groups, hydroxyalkyl ( 3f ), amine ( 3q ), amide ( 3r ), and particularly phenol ( 3g ) and thiophenol groups ( 5u ), were tolerated without the need of protection. The boronic ester group ( 3p ) was compatible to a good degree. Nitroarenes with sterically congested 2,4-xylyl ( 3u ), indane ( 3v ) and naphthyl ( 3w ) groups were also suitable reaction partners. Importantly, nitroheteroarenes could be coupled, giving rise to various heteroaryl amines containing pyrrole ( 4a ), pyrazole ( 4b ), pyridine ( 4c ), quinoline ( 4d ), benzothiophene ( 4e ), benzothiazole ( 4f ), benzoxazole ( 4g ), indole ( 4h, 4i ), indazole ( 4j ) and cuomarin ( 4k ) groups. Notably, unprotected indole ( 4i ) and indazole ( 4j ) were compatible. With respect to the scope of alkyl halides, the reaction protocol allowed the coupling of secondary alkyl iodides with a wide range of acyclic and cyclic substituents, including hydrocarbon groups ( 3a , 3i - 3k, 5a, 5b, 5g , 5j, 5m and 5n ) and functionalized alkyl groups (olefin ( 4f ), ether ( 5c, 5h, 5k ), amine ( 5d ), ester ( 5e ), phthalimide ( 5f ), carbamate ( 5i, 5l )). Both non-activated ( 5o , 5p ) and activated secondary alkyl bromides ( 5q–5t ) reacted to afford the corresponding aryl amines in synthetically useful yields when their loadings were increased to 5 equiv. The introduction of bulky tertiary alkyl groups has been shown to enhance the lipophilicity and metabolic stability of the drugs to improve their potency [23] , [24] . Gratifyingly, tertiary alkyl iodides ( 5u , 5v ) and bromides ( 5w , 5x ) could be coupled using this protocol to give the corresponding N - tert -alkylated amines, albeit with a higher loadings of alkyl halides (4–5 equiv.). Large-scale synthesis (10 mmol) could be achieved without the significant loss in yield (for example, for 3a ). 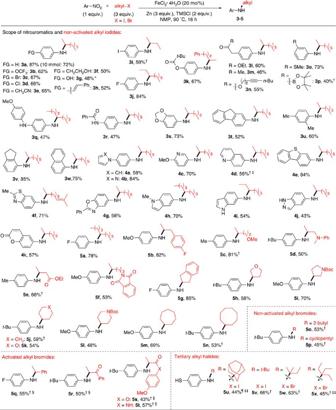Figure 3: Amine synthesis via reductive coupling of nitroarenes with secondary and tertiary alkyl halides. Unless otherwise noted, the optimized conditions were applied; the data are reported as isolated yield. SeeSupplementary Materialsfor experimental details. Boc,tert-butyloxycarbonyl; Bu, butyl; Et, ethyl; Me, methyl; Ph, phenyl;t-Bu,tert-butyl. *RI (2 equiv.);†RI (5 equiv.);‡FeCl2·4H2O (40 mol%), Zn (3.5 equiv.);§FeCl2·4H2O (30 mol%), Zn (3.5 equiv);¶RI (4 equiv.);‡‡FeCl2·4H2O (30 mol %), Zn (4 equiv.). Figure 3: Amine synthesis via reductive coupling of nitroarenes with secondary and tertiary alkyl halides. Unless otherwise noted, the optimized conditions were applied; the data are reported as isolated yield. See Supplementary Materials for experimental details. Boc, tert -butyloxycarbonyl; Bu, butyl; Et, ethyl; Me, methyl; Ph, phenyl; t -Bu, tert -butyl. *RI (2 equiv. ); † RI (5 equiv. ); ‡ FeCl 2 ·4H 2 O (40 mol%), Zn (3.5 equiv. ); § FeCl 2 ·4H 2 O (30 mol%), Zn (3.5 equiv); ¶ RI (4 equiv. ); ‡‡ FeCl 2 ·4H 2 O (30 mol %), Zn (4 equiv.). Full size image Substrate scope of primary alkyl halides Aryl amines substituted with a primary alkyl group are ubiquitous building blocks for biologically active molecules [15] . The N -alkylation of aryl amines with primary alkyl halides is a common method to generate such amines ( Fig. 1b ), but it has a limited scope and may suffer from over-alkylation (see below) [7] . Thus, we sought to apply this reductive coupling method for the coupling of primary alkyl halides. However, the reaction conditions described above were inefficient for the coupling of primary alkyl iodide, as undesired N , N -dialkylaniline was formed in large excess relative to the desired N -alkylaniline ( Supplementary Table 10 , entry 1). A re-optimization showed that reduction of primary alkyl iodide to 1.5 equiv., additions of more Zn (5 equiv.) and TMSCl (4 equiv. ), and lower concentrations of reactants led to a significant suppression of double alkylation ( Supplementary Table 10 , entry 8). Under the new conditions, the coupling of 1a with 1-iodooctane ( 2b ) gave N -octylaniline ( 6a ) and N , N -dioctylaniline ( 7a ) in 76 and 15% GC yields, respectively (compared with 18% 6a and 78% 7a under the protocol in Fig. 3 ) ( Supplementary Table 10 , entries 1 and 8). The modified protocol was applicable for the coupling of a broad range of primary alkyl iodides and bromides ( Fig. 4 ). Both non-functionalized ( 6a – 6c , 6r ) and functionalized alkyl halides ( 6d – 6q ) reacted efficiently to give the target secondary amines in synthetically useful yields, with only a small amount of dialkylation products ( 7a – 7r ). Functional groups such as olefin ( 6d, 6q ), ether ( 6e, 6m ), keto ( 6f ), ester ( 6g, 6n ), amide ( 6h ), nitrile ( 6i ), carbazole ( 6j ), hydroxyl ( 6o ) and chloro moieties ( 6p ) were all tolerated. Molecules containing a bioactive moiety such as menthol ( 6k ) and cholesterol ( 6l ) were compatible as well. The reaction could also be run in a gram scale (10 mmol) with a similar yield (for example, for 6a ). 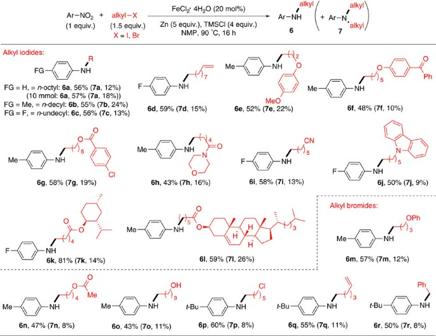Figure 4: Amine synthesis via reductive coupling of primary alkyl halides. Unless otherwise noted, the optimized conditions were applied; the data are reported as isolated yields. SeeSupplementary Materialsfor experimental details. Me, methyl; Ph, phenyl. Figure 4: Amine synthesis via reductive coupling of primary alkyl halides. Unless otherwise noted, the optimized conditions were applied; the data are reported as isolated yields. See Supplementary Materials for experimental details. Me, methyl; Ph, phenyl. Full size image Application To demonstrate its potential utility for medicinal chemistry, this Fe-catalysed amination method was applied for the synthesis of drug-like molecules and their key intermediates. Using this method, N -2-butylaniline 3x , an intermediate to an antiviral agent of human cytomegalovirus ( PD0084430 , 3y ) [25] , was synthesized in a 53% yield ( Fig. 5a ). Subsequent hydrogenolysis of 3x provided the target compound in a 45% overall yield in two steps. Previous method using the reductive amination method gave the product in a lower overall yield (19%) [25] . The amination protocol was also successfully applied for the synthesis of antifungal agents, 5y and 5z (ref. 26 ), giving the product in a single step using commercially available nitroarenes and stable alkyl bromides ( Fig. 5b ). For comparison, the previous reductive amination method required a two-step sequence and involved sensitive Grignard reagents [26] . 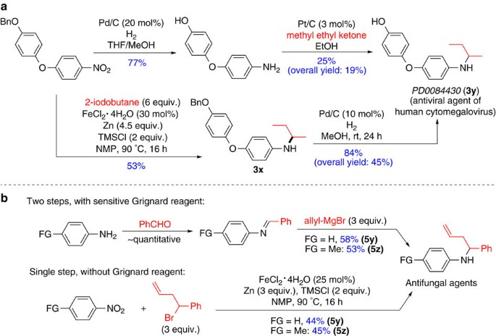Figure 5: Application in medicinal chemistry. (a) Efficient synthesis of the key intermediate of an antiviral agent. (b) Single-step synthesis of antifungal agents. The data are reported as isolated yield. Bn, benzyl; Ph, phenyl. Figure 5: Application in medicinal chemistry. ( a ) Efficient synthesis of the key intermediate of an antiviral agent. ( b ) Single-step synthesis of antifungal agents. The data are reported as isolated yield. Bn, benzyl; Ph, phenyl. Full size image Comparison with direct alkylation and reductive amination Compared with established amination methods such as direct alkylation and reductive amination, the reductive coupling method described here employs a different set of starting materials, which should be advantageous for the synthesis of certain compounds that are difficult using the former methods. This reasoning is supported by examples in Fig. 6 and Supplementary Figs 1–4 (refs 27 , 28 , 29 , 30 ). The direct alkylation of aniline derivative with secondary alkyl halides [28] normally has much lower yields than the reductive coupling ( Fig. 6a,b ; Supplementary Fig. 1 ). Even direct alkylation with a primary alkyl halide [27] might have a much lower yield than the reductive coupling ( Fig. 6c ; Supplementary Fig. 2 ). If an alkyl halide has a functional group susceptible to nucleophilic attack of aniline, for example, 1-bromo-6-chlorohexane, only undesired double alkylation product [31] , but not the desired selective alkylation product, was obtained in 31% yield ( Fig. 6d ). On the contrary, the reductive coupling method gave the desired mono-alkylation product in 52% yield ( Fig. 6d ). Reductive amination using stoichiometric amounts of sodium triacetoxyborohydride (NaBH(OAc) 3 ) proves to be a group-tolerant method for amine synthesis [30] . However, when the ketone or aldehyde reagents contain a keto or alkyl halide functional group, the amination is unsuccessful ( Fig. 6e,f ). On the contrary, the reductive coupling gave the desired amines in synthetically useful yields ( Fig. 6e,f ). 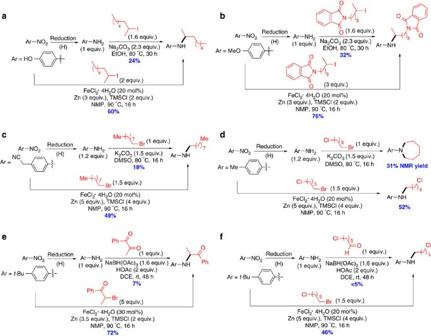Figure 6: Comparison of iron-catalysed reductive coupling method and classical amination methods. (a,b) Comparison with direct alkylation of anilines using secondary alkyl halides. (c,d) Comparison with direct alkylation of anilines using primary alkyl halides. (e,f) Comparison with reductive alkylation. Without otherwise noted, GC yields were reported. DCE, 1,2-dichloroethane; DMSO, dimethyl sulfoxide; EtOH, ethanol; HOAc, acetic acid; Me, methyl; Ph, phenyl;t-Bu,tert-butyl. Figure 6: Comparison of iron-catalysed reductive coupling method and classical amination methods. ( a , b ) Comparison with direct alkylation of anilines using secondary alkyl halides. ( c , d ) Comparison with direct alkylation of anilines using primary alkyl halides. ( e , f ) Comparison with reductive alkylation. Without otherwise noted, GC yields were reported. DCE, 1,2-dichloroethane; DMSO, dimethyl sulfoxide; EtOH, ethanol; HOAc, acetic acid; Me, methyl; Ph, phenyl; t -Bu, tert -butyl. Full size image Mechanistic investigation A number of experiments were conducted to give some insights into the mechanism. In principle, a nitroarene can be reduced by zinc to form an aniline [32] , [33] , which can then undergoes N -alkylation with an alkyl halide to form the alkyl aryl amine product [7] . Indeed, it was found that in the absence of an alkyl halide, 4-nitrotoluene was reduced under the coupling conditions to form 4-methylaniline, albeit in a modest yield ( Fig. 7a ). However, 4-methylaniline did not react with 2-octyl iodide under the coupling conditions to yield the amine product ( Fig. 7a ). Furthermore, under the coupling conditions, the reactions of secondary alkyl iodides with various anilines gave the alkyl amine only in low conversion and yields, while the reductive coupling of nitroarenes with secondary alkyl iodides was efficient ( Supplementary Fig. 5 ). Thus, direct alkylation of in situ formed aniline can be ruled out as the main reaction pathway. 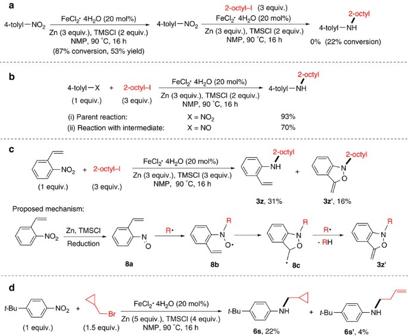Figure 7: Mechanistic study. (a) Reaction of aniline with alkyl halide under the coupling conditions. (b) Comparison of amination reactions using nitroarene and nitrosoarene. (c) Trapping of nitrosoarene intermediate using 2-vinylnitrobenzene as the substrate. (d) Radical-clock experiment using cyclopropylmethyl bromide as the substrate. GC yields were shown inaandb, and isolated yields were shown incandd.t-Bu,tert-butyl. Figure 7: Mechanistic study. ( a ) Reaction of aniline with alkyl halide under the coupling conditions. ( b ) Comparison of amination reactions using nitroarene and nitrosoarene. ( c ) Trapping of nitrosoarene intermediate using 2-vinylnitrobenzene as the substrate. ( d ) Radical-clock experiment using cyclopropylmethyl bromide as the substrate. GC yields were shown in a and b , and isolated yields were shown in c and d . t -Bu, tert -butyl. Full size image Another possible reaction pathway involves the reduction of nitrobenzene by zinc and TMSCl to form nitrosoarene, which subsequently reacts with an alkyl radical generated via iron-mediated reduction of alkyl halide to form the alkyl aryl amine, as described in our initial reaction design ( Fig. 2 ). It was found that 4-methylnitrosobenzene reacted with 2-octyl iodide under the coupling conditions to give the amine product in a 70% yield, while the parent reaction using 4-nitrotoluene had a yield of 93% ( Fig. 7b ). The yields are comparable considering the difference in reagents used. When 2-vinylnitrobenzene was used as a substrate, the expected coupling product ( 3z ) was obtained at the same time as an isoxazole co-product ( 3z′ ) [34] , [35] ( Fig. 7c ). The formation of 3z′ suggests that 2-vinylnitrosobenzene ( 8a ) is generated in the course of reaction. It is proposed that the alkyl radical attacks the nitrogen atom of 8a to form 8b , which undergoes cyclization and hydrogen atom abstraction to give 3z′ . Thus, the above data supports the intermediacy of nitrosoarene as a viable intermediate in the reactions. To further support the involvement of alkyl radicals [36] , 2,2,6,6-tetramethyl-1-piperidinyloxy (TEMPO) was used as a radical trap for the coupling of nitrobenzene with 2-octyl iodide. A significant diminishment in the yield of amination was observed ( Supplementary Fig. 6a ). This result is consistent with the involvement of radicals. When cyclopropylmethyl bromide was used as a radical-clock substrate, both the conventional product ( 6s ) and the ring-opened product ( 6s′ ) were obtained ( Fig. 7d ). This result is again consistent with the formation of alkyl radicals in the coupling reactions. To probe whether alkyl zinc reagent was formed and acted as an intermediate, 2-octyl zinc iodide [37] was treated with nitrobenzene under the coupling conditions, but only a trace of amine product was formed ( Supplementary Fig. 6b ). This result ruled out the intermediacy of alkyl zinc reagents. The present method allows the synthesis of alkyl aryl amines from functionalized nitroarenes, which are often cheaper than functionalized anilines. Moreover, anilines are generally synthesized by reduction of nitroarenes, so amination using directly nitroarenes is more step-economical than using anilines. Additionally, anilines containing easily reducible groups such as alkenes, ketones, and so on would be difficult to obtain by reduction, while the corresponding nitroarenes are readily available and suitable substrates for the current amination ( Fig. 3 ). From these points of view only, the current method can be already considered as a valuable alternative to the conventional amination methods such as direct alkylation and reductive amination. Furthermore, the data in Figs 3 , 4 and 6 , and Supplementary Figs 1–4 also demonstrate potential advantages of the current method in terms of scope, group tolerance, and yield in certain reactions: (i) Our method is applicable for the synthesis of aryl amines substituted with a tertiary alkyl group, of which direct alkylation and reductive amination are incapable ( Supplementary Fig. 3 ). (ii) Direct alkylation using a secondary alkyl halide often has a lower yield than the current method ( Fig. 6a,b ; Supplementary Fig. 1 ). (iii) Direct alkylation using a primary alkyl halide is intolerant to a functional group prone to S N 2 substitution, which is not a problem for the current method as it involves radical alkylation ( Fig. 6d ). (iv) Reductive amination cannot tolerate a keto group or a leaving group prone to S N 2 substitution by aniline, while the current method tolerates well these groups ( Fig. 6e,f ). All in all, our results prove that, despite its early stage of development, the present method exhibits certain potential advantages over the well-established amination methods. The preliminary mechanistic study rules out direct alkylation of in situ formed anilines as a major reaction pathway. The data suggest that alkyl radicals and nitrosoarenes are viable intermediates. The proposed mechanism starts with the reduction of Fe(II) catalyst by Zn to form Fe(I), which activates an alkyl halide to give an alkyl radical. In parallel, Zn reduces nitroarenes to give nitrosoarenes, which is attacked by the alkyl radical to form the C–N bond. The resulting species is then further reduced by Zn and deoxygenated by TMSCl to give the secondary alkyl aryl amine. Consistent with this mechanism, when nitroalkanes were used as substrates, the conversion was full but no amination product was isolated. It is likely that the nitrosoalkane intermediates are less stable than their aryl counterparts and undergo isomerization to give oximes [38] , [39] , [40] , which rapidly dissociate into aldehydes/ketones and hydroxylamine without further reacting with alkyl radical. This mechanism is analogous with the mechanism proposed for the reductive coupling of nitroarenes [14] , [15] , [16] , [17] and nitrite salts [41] with alkenes, which also involves nitroso intermediates. In conclusion, the Fe-catalysed reductive coupling methods presented here represented a general approach to synthesize various (hetero)aryl amines from nitro(hetero)arenes. The ability to couple primary, secondary and tertiary alkyl halides and the high functional group tolerance of the method shall attract applications. Mechanistic study suggests that the addition of an alkyl radical to nitrosoarene is the main reaction pathway. General Supplementary Figs 7–104 for the NMR spectra, Supplementary Tables 1–10 for the optimization of reactions and Supplementary Methods for the characterization data can be found in the Supplementary Information . General procedure for branched alkyl aryl amine synthesis In a nitrogen-filled glove-box, an oven-dried 30 ml re-sealable screw-cap test tube equipped with a Teflon-coated magnetic stir bar was sequentially charged with zinc powder (Zn, 3 equiv. 1.5 mmol), iron(II) chloride tetrahydrate (20 mol%, 0.10 mmol, 20 mg), nitroarene (1 equiv., 0.50 mmol), alkyl iodide (3 equiv., 1.5 mmol), N -methylpyrrolidone solvent (1.0 ml), and chlorotrimethylsilane (3 equiv., 1.5 mmol). The resulting mixture was stirred at 90 °C in a preheated oil bath for 16 h. After the reaction, the reaction mixture was cooled down to room temperature, and the crude product was acidified with saturated NH 4 Cl solution and then neutralized with saturated NaHCO 3 solution. The crude product in the aqueous fraction was extracted with ethyl acetate. The combined organic fractions were concentrated in vacuo with the aid of a rotary evaporator. The crude product residue was purified by flash column chromatography with silica gel using a solvent mixture (ethyl acetate, hexanes) as an eluent to afford the purified amine products ( 3 – 5 ). General procedure for linear alkyl aryl amine synthesis An oven-dried 30 ml re-sealable screw-cap test tube equipped with a Teflon-coated magnetic stir bar was sequentially charged with zinc powder (5 equiv., 2.5 mmol, 164 mg), iron(II) chloride tetrahydrate (20 mol%, 0.10 mmol, 20 mg), nitroarene (1 equiv., 0.50 mmol), primary alkyl iodide (1.5 equiv., 0.75 mmol), N -methylpyrrolidone solvent (2.0 ml), and chlorotrimethylsilane (4 equiv., 2.0 mmol, 128 μl). The resulting mixture was stirred at 90 °C in a preheated oil bath for 16 h. After the reaction, the reaction mixture was cooled down to room temperature, and the crude product was acidified with saturated NH 4 Cl solution and then neutralized with saturated NaHCO 3 solution. The crude product in the aqueous fraction was extracted with ethyl acetate. The combined organic fractions were concentrated in vacuo with the aid of a rotary evaporator. The crude product residue was purified by preparative thin layer chromatography using a solvent mixture (ethyl acetate, hexanes) as an eluent to afford the purified mono-alkylated ( 6 ) and di-alkylated anilines ( 7 ). Data Availability The authors declare that the data supporting the findings of this study are available within the article and its Supplementary Information files . How to cite this article : Cheung, C. W. & Hu, X. Amine synthesis via iron-catalysed reductive coupling of nitroarenes with alkyl halides. Nat. Commun. 7:12494 doi: 10.1038/ncomms12494 (2016).